MHC-I expression renders catecholaminergic neurons susceptible to T-cell-mediated degeneration Subsets of rodent neurons are reported to express major histocompatibility complex class I (MHC-I), but such expression has not been reported in normal adult human neurons. Here we provide evidence from immunolabel, RNA expression and mass spectrometry analysis of postmortem samples that human catecholaminergic substantia nigra and locus coeruleus neurons express MHC-I, and that this molecule is inducible in human stem cell-derived dopamine (DA) neurons. Catecholamine murine cultured neurons are more responsive to induction of MHC-I by gamma-interferon than other neuronal populations. Neuronal MHC-I is also induced by factors released from microglia activated by neuromelanin or alpha-synuclein, or high cytosolic DA and/or oxidative stress. DA neurons internalize foreign ovalbumin and display antigen derived from this protein by MHC-I, which triggers DA neuronal death in the presence of appropriate cytotoxic T cells. Thus, neuronal MHC-I can trigger antigenic response, and catecholamine neurons may be particularly susceptible to T-cell-mediated cytotoxic attack. Antigen presentation requires the expression of major histocompatibility complex (MHC) molecules. This involves the partial intracellular degradation of self and non-self proteins into 8–14 amino acid peptides, loading the peptides to the antigen-binding groove of the MHC class I (MHC-I) or class II (MHC-II), and translocating the complex to the cell surface for display [1] . Although detection of MHC-I in the mature rodent central nervous system (CNS) was for many years confined to glial cells [2] , a body of continuing reports demonstrates that MHC-I can be expressed by some neuronal populations, both in vitro , usually triggered by exposure to interferon gamma (IFN-γ), and in vivo . An initial study showed that MHC-I genes could be induced by IFN-γ in cultured rat hippocampal neurons [3] . Subsequently, mRNA for MHC-I was identified in multiple regions of the neonatal and adult rodent brain including the substantia nigra (SN), brainstem motor neurons (MNs) [4] , the lateral geniculate nucleus (LGN), the cortex, the hippocampus [5] and cerebellum [6] . Subunits of the MHC-I molecule were detected by immunolabel in these regions [7] , [8] , with expression gradually decreasing as neonatal mice reached adulthood in regions including cingulate cortex and the hippocampus [8] . These data suggest a potential role of MHC-I in early development that may be absent in maturity. Neuronal MHC-I expression is thought to play a role in early developmental synaptic plasticity [9] , [10] , [11] , in regeneration of neurons after axotomy [12] and in hippocampus-dependent memory [13] . MHC-I expression has also been shown in cultured hippocampal embryonic neurons that were targeted and killed by CD8 + cytotoxic T cells (CTLs) in response to exogenous viral or ovalbumin (OVA)-derived antigens [14] , [15] . Finally, neurons serve as MHC-I-dependent targets for CTLs following neurotropic viral infections [16] . In humans, MHC-I has been reported in microglia and endothelia of the hippocampus in control individuals and Alzheimer’s disease patients [17] . MHC-II immunolabel of microglia, but not neurons, has been reported in the SN of patients with Alzheimer’s and Parkinson’s disease (PD) [18] , and in the hippocampus of patients with dementia with Lewy bodies [19] . Neuronal expression of MHC-I in the human brain has only been reported in a small number of studies. The first was a study of a childhood viral infection, Rasmussen’s encephalitis, in which immunolabel for the MHC-I component, beta-2-microglobulin (β2m), was present in cortical and hippocampal neurons [20] ; more recently, MHC-I has also been observed in dysmorphic/dysphasic cortical neurons of focal cortical dysplasia, tuberous sclerosis complex and ganglioglioma cases [21] and in the embryonic LGN of the dorsal thalamus [22] and hippocampus [23] . In the LGN, β2m was observed at 29–31 gestational weeks but was nearly absent by postnatal day 55, and was completely absent in the adult [22] . MHC-I in the human visual cortex was not observed at any gestational or postnatal stage [22] , whereas the expression of MHC-I was very low in the hippocampus at 20 gestational weeks and slowly increased during weeks 27–33. A rapid increase in MHC-I molecule expression was found in the subiculum that reached high levels at 31–33 gestational weeks, but no expression of MHC-I was found in the adult hippocampus [23] . To date, there has been no evidence reported of neuronal MHC-I expression in the normal adult human brain. In this study, we show that in human postmortem samples from adult control individuals and PD patients, MHC-I is expressed by SN dopaminergic (DA) and locus coeruleus (LC) norepinephrinergic (NE) neurons; the proportion of catecholamine locus coeruleus neurons that express MHC-I in humans is higher in controls than in PD subjects; human stem cell (hES)- in vitro -derived DA neurons can be induced to express MHC-I in their membranes; catecholamine murine neurons in primary culture are more prone to display MHC-I upon IFN-γ challenge than non-catecholamine neurons; SN DA murine neurons in culture display MHC-I in response to microglia activated by neuromelanin (NM) or alpha-synuclein (α-syn), substances found extracellularly in postmortem PD brain; in the absence of microglia, chronic exposure to the DA precursor, L-dihydroxyphenylalanine (L-DOPA), induces MHC-I in SN DA murine neurons; SN murine neurons in culture can process and present foreign protein antigens by MHC-I; in the presence of the appropriate antigen and CTLs, MHC-I expressing SN murine neurons are destroyed. These findings suggest that neuronal MHC-I expression and antigen display in catecholamine neurons may be triggered by microglial activation or high cytosolic DA, which in the presence of the appropriate antigen and CTLs could play a role in neuronal death during diseases in which CNS inflammation is robust. MHC-I in human catecholamine neurons Human MHC-I consists of an α-chain encoded by HLA genes (HLA-A, HLA-B and HLA-C) and a noncovalently associated β2m subunit. We used a variety of techniques to assess the presence of MHC-I in human postmortem samples. First, we examined MHC-I expression by immunofluorescence using a primary antibody against human HLA α-chain (amino acids 63–362) that detects an epitope common in HLA-A, B and C, together with an antibody against Fox-3, a neuronal nuclei marker. We initially examined sections of hippocampus with adjacent entorhinal cortex from human controls (59–85 years old). Consistent with previous reports, blood vessels in hippocampus and cortex were labelled for HLA, and we did not observe any label in neurons or glia ( Fig. 1a ). MHC-II was never observed in neurons. Similarly, HLA immunolabel in sections of the caudate nucleus from control postmortem samples in the same age range was observed only in blood vessels, and not in glia or neurons ( Fig. 1a ). 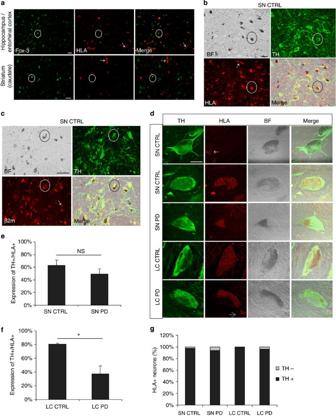Figure 1: Human SN and LC express MHC-I. (a) Fluorescent images showing double immunolabel for the neuronal nuclei marker, Fox-3 (green) and human MHC-I HLA (A, B and C, red) in human postmortem hippocampal/entorhinal cortex sections and striatal sections from control individuals. White circles demonstrate that there is no overlap between neurons and HLA+structures. Scale bar, 60 μm. (b,c) Brightfield and immunofluorescence images of SN stained for (b) HLA (A, B and C, red) and TH (green) and (c) β2m (red) and TH (green). NM was identified under brightfield illumination. Encircled neurons demonstrate that TH+neurons display HLA immunolabel, overlapping in particular with NM. Scale bar, 50 μm inband 75 μm inc100 μm. (d) Confocal immunofluorescent label of TH (green) and HLA (A, B and C, red) in SN and LC control and PD samples. The first row shows a representative example of an SN DA neuron that does not express HLA. When HLA was observed in SN and LC neurons (examples in the second through fifth rows), it was often associated with NM. Scale bar, 25 μm. (eandf) Proportion of TH+neurons with HLA (A, B and C) immunolabel in the SN (e) and the LC (f). Cell counts were performed in three sections per brain of eight control individuals and eight PD patients (SN) and eight control individuals and nine PD patients (LC). Data are presented as the mean±s.e.m.P>0.05 (NS) in E (Mann–WhitneyU-test) and *P<0.05 in F (Mann–WhitneyU-test). (g) Percentage of TH+and TH−neurons in the SN and LC (control and PD) labelled for HLA. The arrows in all panels point to blood vessels. Each experiment was repeated at least in triplicate. BF, brightfield; CTRL, control; NS, nonsignificant. Figure 1: Human SN and LC express MHC-I. ( a ) Fluorescent images showing double immunolabel for the neuronal nuclei marker, Fox-3 (green) and human MHC-I HLA (A, B and C, red) in human postmortem hippocampal/entorhinal cortex sections and striatal sections from control individuals. White circles demonstrate that there is no overlap between neurons and HLA + structures. Scale bar, 60 μm. ( b , c ) Brightfield and immunofluorescence images of SN stained for ( b ) HLA (A, B and C, red) and TH (green) and ( c ) β2m (red) and TH (green). NM was identified under brightfield illumination. Encircled neurons demonstrate that TH + neurons display HLA immunolabel, overlapping in particular with NM. Scale bar, 50 μm in b and 75 μm in c 100 μm. ( d ) Confocal immunofluorescent label of TH (green) and HLA (A, B and C, red) in SN and LC control and PD samples. The first row shows a representative example of an SN DA neuron that does not express HLA. When HLA was observed in SN and LC neurons (examples in the second through fifth rows), it was often associated with NM. Scale bar, 25 μm. ( e and f ) Proportion of TH + neurons with HLA (A, B and C) immunolabel in the SN ( e ) and the LC ( f ). Cell counts were performed in three sections per brain of eight control individuals and eight PD patients (SN) and eight control individuals and nine PD patients (LC). Data are presented as the mean±s.e.m. P >0.05 (NS) in E (Mann–Whitney U -test) and * P <0.05 in F (Mann–Whitney U -test). ( g ) Percentage of TH + and TH − neurons in the SN and LC (control and PD) labelled for HLA. The arrows in all panels point to blood vessels. Each experiment was repeated at least in triplicate. BF, brightfield; CTRL, control; NS, nonsignificant. Full size image We then performed double immunolabeling for HLA and Fox-3, or HLA and the catecholamine marker tyrosine hydroxylase (TH), in the SN and LC of control and PD samples. In sharp contrast to the other brain regions examined, HLA immunolabel was present selectively in many of the TH + NM-containing neurons, as well as blood vessels ( Fig. 1b and Supplementary Fig. 1 ). We independently confirmed the presence of MHC-I in SN neurons by double immunofluorescence label for TH and an antibody against amino acids 1–120 of human β2m, the β-chain component of MHC-I ( Fig. 1c ). The β2m cellular distribution and neuronal pattern of staining appeared identical to that of the HLA α-chain (compare Fig. 1b,c ). Immunolabel for both MHC-I components was observed throughout the cytosol and often at particularly high levels in regions associated with NM in both SN and LC catecholamine neurons ( Fig. 1b,c,d and Supplementary Fig. 1 ). The specificity of the neuronal MHC-I immunolabel was confirmed by the absence of staining when the respective primary antibodies were pre-adsorbed by recombinant HLA or β2m peptides (see Methods). In SN postmortem material from eight control individuals, 62.53±8.6% (mean±s.e.m.) of TH + neurons displayed HLA + label, whereas 49.03±8.7% (mean±s.e.m.) were labelled in eight age-matched PD patients ( Fig. 1e ). Only <3% of TH − SN control neurons and <7% of TH − SN PD patient neurons expressed HLA ( Fig. 1g ). In the same sections, we observed no DA neurons in the ventral tegmental area (VTA) that expressed MHC-I ( Supplementary Fig. 2A ). In the LC, 80.3±1.8% (mean±s.e.m.) of TH + neurons were HLA + from eight control individuals, and 37.3±11.8% of TH + were HLA + in neurons of nine age-matched PD patients; this difference was statistically significant ( Fig. 1f ). No TH − neurons expressed HLA label in LC control samples, and less than 5% TH − did in LC PD ( Fig. 1g ). We used multiple approaches to corroborate the identification of MHC-I in SN neurons obtained by immunofluorescence. To discard artifacts due to autofluorescence, we assessed the presence of MHC-I via immunoperoxidase label. HLA label was clearly present in blood vessels, and negligible in microglia, astrocytes and NM − neurons ( Supplementary Fig. 2B ). In contrast, we observed clear HLA immunoperoxidase label in NM + SN and LC neurons, both in control and in PD samples ( Fig. 2a ). MHC-II was never observed in neurons. We then examined HLA immunolabel in LC and SN from control samples by immunoelectron microscopy. Consistent with the immunofluorescent images of MHC-I, immunogold label for MHC-I was associated with blood vessels and was clearly present in NM organelles in LC and SN neurons ( Fig. 2b , Supplementary Fig. 2C ). 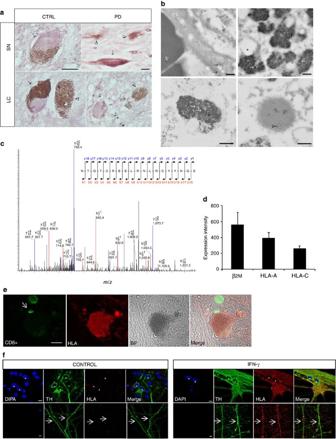Figure 2: Human SN and LC express MHC-I with local CTLs. (a) V-VIP immunostain (purple) indicates HLA (A, B and C) in control and PD SN and LC samples. NM appears as brown precipitate. Arrows indicate labelled cells in which the chromogen fills and outlines cell bodies and occasional dendrites. The arrowheads indicate NM+neurons devoid of cytosolic immunocytochemical label. Scale bar, 25 μm in the left panels and 15 μm in the right panels. (b) Immunoelectron microscopy images demonstrating antigenicity to HLA (A, B and C) within NM granules of control SN and LC (white arrows). Blood vessel endothelium was used as a positive control for the HLA antibody and showed immunolabel (black arrows); the erythrocyte showed very little staining (white outlined arrowhead). Lipid bodies (asterisk) within NM organelles did not exhibit HLA immunolabel. The black outlined arrowhead depicts a lysosome with HLA label in an LC neuron. Scale bar, 250 nm. (c) MS/MS spectrum (parent ionm/z788.2=[M+3H]3+) corresponding to the peptide NTQTDRESLRNLRCYYNQS observed in the analysis of NM isolated from SN tissue. SeeTable 1for details. (d) β2m, HLA-A and HLA-C genes are robustly expressed in laser-captured NM SN neurons of control individuals. Data are presented as the mean±s.e.m. Samples from 9 control subjects were analyzed. (e) Double immunofluorescence in the SN of human of a postmortem control sample. NM was observed under brightfield microscopy. An arrow indicates a CD8+T-cell in contact with a NM+neuron. Scale bar, 15 μm. (f) Immunofluorescence in hES-derived DA neurons, showing HLA (A, B and C) immunolabel in the cell body (upper panel) and dendrites (lower panel) of TH+neurons exposed to human IFN-γ, but not in neurons treated with the vehicle. Asterisks indicate cell bodies and arrows point at dendrites. Scale bar, 10 μm. Each experiment was repeated at least in triplicate, and within each experiment, each condition was also performed at least three times. BF, brightfield; CTRL, control. Figure 2: Human SN and LC express MHC-I with local CTLs. ( a ) V-VIP immunostain (purple) indicates HLA (A, B and C) in control and PD SN and LC samples. NM appears as brown precipitate. Arrows indicate labelled cells in which the chromogen fills and outlines cell bodies and occasional dendrites. The arrowheads indicate NM + neurons devoid of cytosolic immunocytochemical label. Scale bar, 25 μm in the left panels and 15 μm in the right panels. ( b ) Immunoelectron microscopy images demonstrating antigenicity to HLA (A, B and C) within NM granules of control SN and LC (white arrows). Blood vessel endothelium was used as a positive control for the HLA antibody and showed immunolabel (black arrows); the erythrocyte showed very little staining (white outlined arrowhead). Lipid bodies (asterisk) within NM organelles did not exhibit HLA immunolabel. The black outlined arrowhead depicts a lysosome with HLA label in an LC neuron. Scale bar, 250 nm. ( c ) MS/MS spectrum (parent ion m / z 788.2=[M+3H] 3+ ) corresponding to the peptide NTQTDRESLRNLRCYYNQS observed in the analysis of NM isolated from SN tissue. See Table 1 for details. ( d ) β2m, HLA-A and HLA-C genes are robustly expressed in laser-captured NM SN neurons of control individuals. Data are presented as the mean±s.e.m. Samples from 9 control subjects were analyzed. ( e ) Double immunofluorescence in the SN of human of a postmortem control sample. NM was observed under brightfield microscopy. An arrow indicates a CD8 + T-cell in contact with a NM + neuron. Scale bar, 15 μm. ( f ) Immunofluorescence in hES-derived DA neurons, showing HLA (A, B and C) immunolabel in the cell body (upper panel) and dendrites (lower panel) of TH + neurons exposed to human IFN-γ, but not in neurons treated with the vehicle. Asterisks indicate cell bodies and arrows point at dendrites. Scale bar, 10 μm. Each experiment was repeated at least in triplicate, and within each experiment, each condition was also performed at least three times. BF, brightfield; CTRL, control. Full size image As NM organelles can be efficiently isolated from human SN [24] , [25] , mass spectrometry was used to detect the presence of MHC proteins in isolated NM organelles and purified NM. A variety of MHC-I components, including peptides corresponding to alleles of HLA-A, HLA-B, HLA-C and β2m genes ( Fig. 2c , Table 1 ) were detected in both NM organelles and purified NM; in contrast, no MHC-II peptides were identified in any human SN NM sample. Table 1 MHC-I peptides associated with NM and identified by mass spectrometry analysis of samples isolated from human SN. Full size table We also evaluated the abundance of MHC-I mRNA in human NM + SN neurons from control samples. Robust expression signals were confirmed for the β2M and HLA-A and HLA-C genes in a laser-captured NM SN neuron microarray data set 26 , comprising nine ( Fig. 2d ) control individuals without neurodegenerative diseases (mean age at death (range), 75 years (61–80). It is impossible to determine if neuronal MHC-I in postmortem tissue was immunologically competent, but the presence of CTLs in SN and LC would indicate that such interactions could occur. CD8 + and CD4 + cells have been identified previously in human SN in close vicinity to NM + neurons, and are present at particularly high levels in PD [27] . Using double immunolabel for HLA and CD8 + CTLs in SN and LC samples, we sometimes observed CD8 + CTLs in close proximity to HLA-expressing NM + neurons in both control ( Fig. 2e ) and PD specimens ( Supplementary Fig. 2D ); in some cases, catecholaminergic HLA + neurons and CTLs appeared to be in contact ( Fig. 2e ). MHC-I induction hES-derived DA neurons CNS neurons in postmortem samples do not retain intact plasma membranes. To confirm that MHC-I can be localized in the plasma membrane of human DA neurons, we examined neuronal cultures derived from hES that exhibit a range of properties of SN DA neurons [28] . Mature midbrain DA neurons (150 days in culture) displayed a dense TH + fibre network that extended over distances of several millimetres. IFN-γ is a proinflammatory cytokine found at high levels in cerebrospinal fluid and blood of patients with neurodegenerative disorders [29] that induces MHC-I expression in antigen-presenting cells by activating a regulatory element of the MHC-I promoter [30] . Untreated DA neurons exhibited no MHC-I; however, human IFN-γ induced plasma membrane expression of MHC-I by virtually all TH + neurons ( Fig. 2f ). In control experiments to assess neuronal specificity, mature MNs derived from hES were examined after exposure to human IFN-γ, but no MHC-I expression was observed ( Supplementary Fig. 3A ). Induction of neuronal MHC-I in murine catecholamine neurons To study the mechanisms underlying the preferential display of MHC-I by catecholamine neurons, we examined primary neuronal cultures of >7 days in vitro prepared from 0–3 day old C57BL/6 mice [31] . DA neurons from VTA and SN and NE neurons of the LC were identified by immunolabel for TH. We examined MHC-I staining using an antibody raised against the H-2K b and H-2D b class I mouse alloantigens. Untreated TH + neurons exhibited no MHC-I immunolabel ( Fig. 3a ). We then examined the response to recombinant mouse IFN-γ, which induced robust plasma membrane neuronal MHC-I expression on TH + neurons ( Fig. 3a ; Supplementary Movie 1 ). 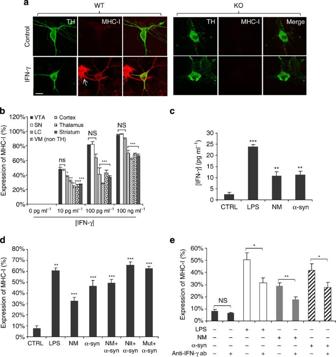Figure 3: Induced MHC-I by murine catecholamine neurons. (a) MHC-I immunolabel in postnatally-derived cultured SN DA neurons from wild-type and β2m KO mice imaged by confocal microscopy. The upper row shows untreated DA (TH: green) neurons. The bottom row shows MHC-I (red) expressing DA neurons exposed to IFN-γ. The arrow indicates a MHC-I expressing astrocyte (bottom row). Scale bar, 20 μm. (b) Dose response of MHC-I induction by IFN-γ in neurons obtained from various brain regions. Data are presented as the mean±s.e.m. (NS; **P<0.01; ***P<0.001, Two-way analysis of variance (ANOVA) test). (c) IFN-γ released by microglia stimulated with LPS, NM or α-syn. Data are presented as the mean±s.e.m. (**P<0.01; ***P<0.001, one-way ANOVA with Tukeypost hoctest). (d) Expression of MHC-I after exposing primary VM neurons to medium from microglia pre-stimulated with LPS, NM or α-syn (wild type, nitrated or A53T mutant). Data are presented as the mean±s.e.m. (*P<0.05; **P<0.01; ***P<0.001, one-way ANOVA with Tukeypost hoctest). (e) Percentage of VM neurons that expressed MHC-I after exposure to microglial condition as in (c), with or without a neutralizing antibody for IFN-γ. Data are presented as the mean±s.e.m. (NS; *P<0.05; **P<0.01, two-tailed Student’st-test). Each experiment was repeated at least in triplicate, and within each experiment, each condition was also performed at least three times. For each condition, neurons onn=24 fields at × 20 were quantified. ab, antibody; CTRL, control; NS, nonsignificant; WT, wild type. Figure 3: Induced MHC-I by murine catecholamine neurons. ( a ) MHC-I immunolabel in postnatally-derived cultured SN DA neurons from wild-type and β2m KO mice imaged by confocal microscopy. The upper row shows untreated DA (TH: green) neurons. The bottom row shows MHC-I (red) expressing DA neurons exposed to IFN-γ. The arrow indicates a MHC-I expressing astrocyte (bottom row). Scale bar, 20 μm. ( b ) Dose response of MHC-I induction by IFN-γ in neurons obtained from various brain regions. Data are presented as the mean±s.e.m. (NS; ** P <0.01; *** P <0.001, Two-way analysis of variance (ANOVA) test). ( c ) IFN-γ released by microglia stimulated with LPS, NM or α-syn. Data are presented as the mean±s.e.m. (** P <0.01; *** P <0.001, one-way ANOVA with Tukey post hoc test). ( d ) Expression of MHC-I after exposing primary VM neurons to medium from microglia pre-stimulated with LPS, NM or α-syn (wild type, nitrated or A53T mutant). Data are presented as the mean±s.e.m. (* P <0.05; ** P <0.01; *** P <0.001, one-way ANOVA with Tukey post hoc test). ( e ) Percentage of VM neurons that expressed MHC-I after exposure to microglial condition as in ( c ), with or without a neutralizing antibody for IFN-γ. Data are presented as the mean±s.e.m. (NS; * P <0.05; ** P <0.01, two-tailed Student’s t -test). Each experiment was repeated at least in triplicate, and within each experiment, each condition was also performed at least three times. For each condition, neurons on n =24 fields at × 20 were quantified. ab, antibody; CTRL, control; NS, nonsignificant; WT, wild type. Full size image Detection of MHC-I immunolabel can be influenced by fixation, and therefore we also examined labelling of living neurons. Immunolabel for MHC-I was absent in control neuronal cultures and was observed in unfixed neurons only following IFN-γ ( Supplementary Fig. 3B ), indicating that detection of neuronal MHC-I was not an artifact of fixation. To confirm that the immunolabel was specific for MHC-I, we examined neurons cultured from MHC-I null (‘knockout’: KO) mice that are deficient for β2m (B6.129P2-B2mtm1Unc/J). As expected, IFN-γ did not induce MHC-I (H-2Kb and H-2Db) immunolabel in the mutant neurons ( Fig. 3a ). We further conducted a series of control experiments in which we examined wild-type and KO astrocytes combinatorially with wild-type and KO neurons. For each combination, wild-type neurons and astrocytes were induced to express MHC-I by IFN-γ, whereas in each case the KO neurons and astrocytes never expressed MHC-I. We compared the response to IFN-γ by LC and ventral midbrain (VM: SN and VTA) catecholamine neurons to cortical, thalamic, striatal and non-DA SN-cultured neurons that were identified by label for the neuron-specific cytoskeleton protein, microtubule-associated protein-2 (MAP-2). Catecholamine neurons of the SN, VTA and LC were far more responsive to IFN-γ than were non-catecholamine neurons: even 1,000-fold excesses of IFN-γ did not induce non-catecholamine neurons to express MHC-I at the level of catecholamine neurons (compare 100 pg ml −1 to 100 ng ml −1 , Fig. 3b ). Regulation of MHC-I expression by activated microglia The induction of MHC-I in our SN neuronal culture experiments, as well as in prior reports from other neurons [14] , [15] , was triggered by IFN-γ. This cytokine is considered to be a product of lymphoid cells, but CNS microglia provide an alternate source of this proinflammatory signal [32] . Activated microglia have long been recognized in a variety of neurodegenerative disorders, including PD [33] . Extracellular NM, which is a remnant of dead SN neurons [33] , and various forms of extracellular α-syn can activate microglia [34] , [35] . Using an enzyme-linked immunosorbent assay (ELISA), we found that primary microglial cultures exposed to human NM or native α-syn for 72 h secreted 5–10-fold more IFN-γ than untreated cells ( Fig. 3c ). Control experiments revealed that lipopolysaccharide (LPS), an inflammatory component from Gram-negative bacteria, also induced IFN-γ secretion in primary microglial culture ( Fig. 3c ). Both overexpression and multiple mutations of α-syn are implicated in PD [36] , [37] . We examined the effects of conditioned media from microglial cultures exposed to NM or a variety of modified α-syn proteins on neuronal MHC-I expression. The conditioned medium obtained from microglia cultures incubated for 72 h with NM, α-syn, NM with α-syn, nitrated α-syn (Nit-α-syn), A53T mutant α-syn (Mut-α-syn) or LPS, elicited cell surface MHC-I presentation by VM neurons ( Fig. 3d ). This induction of MHC-I expression was in part mediated by IFN-γ, as the addition of IFN-γ neutralizing antibody to the conditioned medium decreased MHC-I expression by 30–50% ( Fig. 3e ). In contrast, there was no induction of neuronal MHC-I when cultures were directly exposed to equivalent levels of LPS, α-syn or NM in the absence of microglial cells. These results indicate that substances including NM and α-syn can activate microglia, as demonstrated by the release of IFN-γ, as well as that additional inflammatory factors induce MHC-I display by VM neurons. Primary cortical and striatal neurons were also analyzed for MHC-I expression after exposure to microglial medium pre-incubated for 72 h with LPS, NM or α-syn under the same conditions used for VM DA cultures. Under these conditions, cortical and striatal neurons also expressed MHC-I, but at a significantly lower proportion than VM DA neurons ( Supplementary Fig. 3C ). Regulation of MHC-I expression by oxidative stress Protein oxidation has been suggested to provide a ‘global signal’ that induces MHC-I expression [38] . DA-derived oxidative stress has been associated with neurodegenerative diseases including PD [39] , in part because cytosolic DA, which is also the precursor to NE in LC neurons, can be metabolized to a quinone that reacts with proteins including α-syn [40] , [41] . DA-modified α-syn leads to cellular toxicity and autophagy dysfunction [42] , [43] . Moreover, oxidation of cytosolic DA triggers NM synthesis as an autophagic cellular stress response [24] . We thus hypothesized that conditions that promote oxidative stress via high cytosolic DA [44] may account for the selectivity of neuronal MHC-I expression by catecholamine neurons. To enhance cytosolic DA, we used the DA precursor, L-DOPA, which is accumulated by amino acid transport and converted into DA in the cytosol. Exposure to high levels of L-DOPA can produce NM in both catecholaminergic and nominally non-catecholaminergic cells [24] . L-DOPA is used therapeutically in PD treatment, and while there is no clear evidence indicating that L-DOPA is toxic in humans including PD patients, the compound can be toxic to cultured cells [44] , [45] . We exposed SN murine neuronal cultures to L-DOPA under conditions that substantially increase cytosolic DA as measured by intracellular patch electrochemistry [44] and promote NM production as observed by brightfield microscopy [24] . Control SN neurons exhibited no visible NM, whereas the addition of L-DOPA induced NM in 40% of the neurons ( Fig. 4a,b ), confirming the formation of non-degradable oxidized catecholamine products within autophagic organelles [24] . We found that L-DOPA stimulated neuronal MHC-I display in ~10% of TH + neurons and ~7% of TH − neurons ( Fig. 4c ). 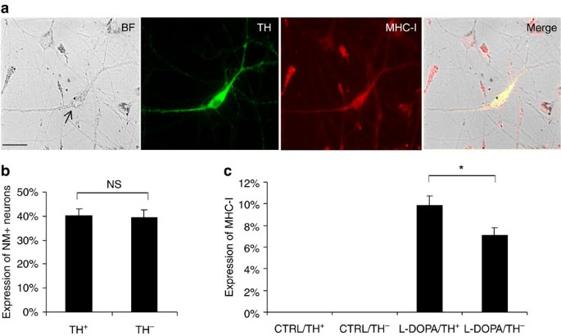Figure 4: MHC-I induction in VM DA neurons is dependent on oxidative stress. (a) Example of TH/MHC-I double immunolabel of primary cultures of VM neurons after treatment with L-DOPA, which induced the presence of both NM (arrow) and MHC-I. Scale bar, 30 μm. (b) Fraction of TH+and TH−neurons that displayed NM following L-DOPA. Data are presented as mean±s.e.m. (NS, two-tailed Student’st-test). (c) The fraction of TH+and TH−neurons that displayed plasma membrane MHC-I following L-DOPA. Data are presented as mean±s.e.m. (*P<0.05, two-tailed Student’st-test). Each experiment was repeated at least in triplicate and within each experiment, each condition was also performed at least three times. For each condition, neurons onn=24 fields at × 20 were quantified. BF, brightfield; CTRL, control; NS, nonsignificant. Figure 4: MHC-I induction in VM DA neurons is dependent on oxidative stress. ( a ) Example of TH/MHC-I double immunolabel of primary cultures of VM neurons after treatment with L-DOPA, which induced the presence of both NM (arrow) and MHC-I. Scale bar, 30 μm. ( b ) Fraction of TH + and TH − neurons that displayed NM following L-DOPA. Data are presented as mean±s.e.m. (NS, two-tailed Student’s t -test). ( c ) The fraction of TH + and TH − neurons that displayed plasma membrane MHC-I following L-DOPA. Data are presented as mean±s.e.m. (* P <0.05, two-tailed Student’s t -test). Each experiment was repeated at least in triplicate and within each experiment, each condition was also performed at least three times. For each condition, neurons on n =24 fields at × 20 were quantified. BF, brightfield; CTRL, control; NS, nonsignificant. Full size image Altogether, our data indicate that high levels of neuronal DA can induce the formation of pigmented NM organelles and the presentation of neuronal MHC-I even in the absence of microglia or exogenously added IFN-γ. This suggests that redox stress in neuronal cytosol due to cytosolic catecholamines could underlie the particular expression of MHC-I by catecholamine neurons. This is also consistent with the observation that TH − neurons can display MHC-I when treated with L-DOPA, which induces accumulation of catechols in cytosol followed by their subsequent oxidation. We note that L-DOPA exposure in patients is substantially lower than in our culture system, and may not be sufficient to enhance oxidation or MHC-I display, but our findings suggest that a history of cytosolic catecholamine could underlie the MHC-I display specific to catecholamine neurons in adult human. SN neurons are antigen-presenting cells A characteristic of ‘professional’ antigen cells such as dendritic cells (DCs) is their capacity to process and load antigen onto the MHC-I groove. Although previous in vitro studies show hippocampal neurons display MHC-I upon exposure to IFN-γ and present small peptides exogenously added to the culture [14] , [15] , there are to our knowledge no reports examining whether neurons can internalize, process and load antigens onto MHC-I as other cells do. To examine antigen presentation by cultured neurons, we removed all sources of BSA from the media, and exposed VM neuronal cultures to chicken OVA. OVA is a 385 amino acid foreign protein that can be cleaved to an eight amino acid SIINFEKL peptide by DCs and other ‘professional’ antigen-presenting cells; the SIINFEKL peptide is then loaded and presented in their MHC-I groove [46] . Following exposure of SN neuronal cultures to OVA or vehicle for 7 days, neurons were exposed to IFN-γ or saline for 72 h (note that these cultures were never exposed to SIINFEKL). We then double immunolabeled our cultures for TH and an antibody that recognizes the MHC-I complex only when occupied by SIINFEKL (SIINFEKL-MHC-I). Occasional label of astrocytes, but not neurons, for SIINFEKL-MHC-I was observed when the cultures were exposed to the vehicle, IFN-γ or OVA alone ( Fig. 5a ). In contrast, ~10% of TH + neurons exposed to both OVA and IFN-γ were immunolabeled for SIINFEKL-MHC-I ( P <0.001, one-way ANOVA (analysis of variance); Fig. 5b ) that was present throughout the cytoplasm, indicating that SIINFEKL was loaded onto MHC-I within the neuron. In contrast, when cultures were exposed to IFN-γ with extracellular SIINFEKL as a positive control, ~70% of TH + neurons exhibited SIINFEKL-MHC-I immunolabel selectively on the plasma membrane and not in the cytosol ( P <0.001, one-way ANOVA, Fig. 5a,b ). Our results indicate that OVA had been processed to SIINFEKL within these mixed neuron/astrocyte cultures and loaded into the MHC-I groove within neuronal cytosol, and that the resulting complex was presented on the neuronal plasma membrane. 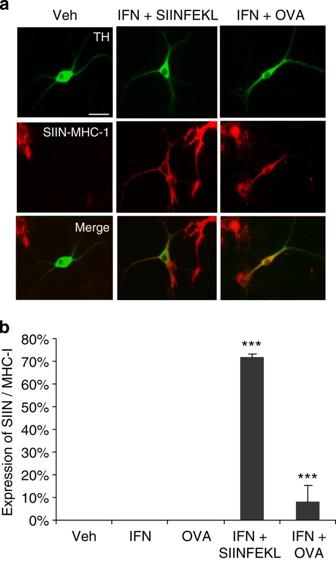Figure 5: VM DA neurons load and display antigen. (a) VM DA neurons immunolabeled for TH and SIINFEKL-MHC-I. (b) The fraction of TH+neurons that were labelled for SIINFEKL-MHC-I following vehicle, IFN-γ, OVA, IFN-γ+SIINFEKL and IFN-γ+OVA. Data are presented as the mean±s.e.m. (***P<0.001, one-way analysis of variance with Tukeypost hoctest). Each experiment was repeated at least in triplicate and within each experiment, each condition was also performed at least three times. For each condition, neurons onn=24 fields at × 20 were quantified. Scale bar, 30 μm. IFN, interferon gamma; SIIN, SIINFEKL; Veh, vehicle. Figure 5: VM DA neurons load and display antigen. ( a ) VM DA neurons immunolabeled for TH and SIINFEKL-MHC-I. ( b ) The fraction of TH + neurons that were labelled for SIINFEKL-MHC-I following vehicle, IFN-γ, OVA, IFN-γ+SIINFEKL and IFN-γ+OVA. Data are presented as the mean±s.e.m. (*** P <0.001, one-way analysis of variance with Tukey post hoc test). Each experiment was repeated at least in triplicate and within each experiment, each condition was also performed at least three times. For each condition, neurons on n =24 fields at × 20 were quantified. Scale bar, 30 μm. IFN, interferon gamma; SIIN, SIINFEKL; Veh, vehicle. Full size image VM DA neuronal killing by CTLs We first examined the capacity of CTLs to respond to MHC-I induced SN neurons by following CTL proliferation using BrdU (5-bromo-2'-deoxyuridine) incorporation. We compared the induction of CTL proliferation by DCs and VM neuronal cultures using OT-1 CTL cells that constitutively recognize and respond to SIINFEKL [47] , and found that the combination of IFN-γ and SIINFEKL induced similar CTL proliferation by both DC and VM neuronal cultures ( Supplementary Fig. 3D ). In contrast, we observed no neuronally induced proliferation of another clonal CD4 + T-cell line that specifically recognizes MHC-II. These results led us to examine whether neuronal antigen-loaded MHC-I was competent to trigger CTL-mediated cell death. We used the OT-1 CTL line as effector cells [47] and SIINFEKL peptide-pulsed SN neurons as target cells. The combination of CTLs, IFN-γ and SIINFEKL killed 55% of TH+ neurons; as expected, no neuronal death was triggered in similarly treated cultures of MHC-I null (knockout: KO) SN neurons ( Fig. 6a ). The presence of CTLs was required to elicit neuronal death, as medium conditioned by SIINFEKL-activated CTLs but with the CTLs themselves omitted, did not kill neurons ( Supplementary Fig. 3E ). To determine whether the astrocyte monolayer played a role in the CTL-mediated neuronal death, we compared cultures in which wild-type or KO astrocytes were plated under wild-type ventral midbrain neurons. MHC-I was induced by IFN-γ, and then SIINFEKL and OT-1 cells were added to the culture. We did not observe different levels of neuronal death between neurons plated on wild-type astrocytes or KO astrocytes, indicating that the ability of astrocytes in culture to express MHC-I is irrelevant to OT-1-mediated neuronal death ( Supplementary Fig. 3F ). 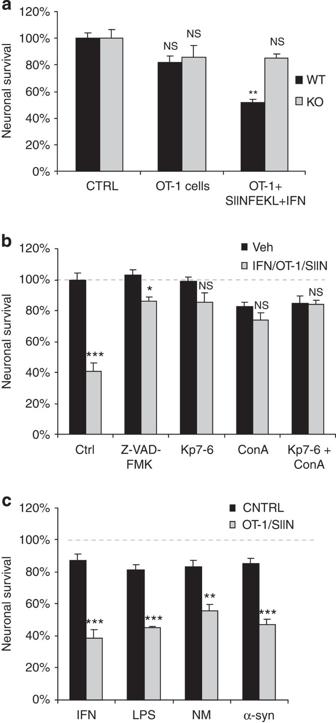Figure 6: VM DA neurons that display antigen are killed by CD8+ T cells. (a) The fraction of VM DA neurons surviving in the presence of SIINFEKL, OT-1 cells pre-pulsed with SIINFEKL, and IFN-γ (100 ng ml−1) in cultures obtained from wild-type and β2m KO mice. Data are presented as the mean±s.e.m. (NS; **P<0.01, One-way analysis of variance (ANOVA) with Tukeypost hoctest). (b) Survival of VM DA neurons incubated with IFN-γ, SIINFEKL peptide and OT-1 cells with the pan-caspase inhibitor Z-VAD-FMK, the Fas/Fas ligand antagonist, Kp7-6, the perforin/granzyme antagonist, concanamycin A or the combination of Kp7-6 and concanamycin A. Data are presented as the mean±s.e.m. (NS; *P<0.05, ***P<0.001, one-way ANOVA with Tukeypost hoctest). (c) VM DA neuron survival with SIINFEKL, OT-1 cells pre-pulsed with SIINFEKL and microglial medium previously exposed to LPS, α-syn or NM. Data are presented as the mean±s.e.m. (NS; *P<0.05, **P<0.01; ***P<0.001, one-way ANOVA with Tukeypost hoctest). Each experiment was repeated at least in triplicate and within each experiment, each condition was also performed at least three times. For each condition, neurons onn=24 fields at × 20 were quantified. ConA, concanamycin A; CTRL, control; IFN, interferon gamma; NS, nonsignificant; SIIN, SIINFEKL; Veh, vehicle. Figure 6: VM DA neurons that display antigen are killed by CD8+ T cells. ( a ) The fraction of VM DA neurons surviving in the presence of SIINFEKL, OT-1 cells pre-pulsed with SIINFEKL, and IFN-γ (100 ng ml −1 ) in cultures obtained from wild-type and β2m KO mice. Data are presented as the mean±s.e.m. (NS; ** P <0.01, One-way analysis of variance (ANOVA) with Tukey post hoc test). ( b ) Survival of VM DA neurons incubated with IFN-γ, SIINFEKL peptide and OT-1 cells with the pan-caspase inhibitor Z-VAD-FMK, the Fas/Fas ligand antagonist, Kp7-6, the perforin/granzyme antagonist, concanamycin A or the combination of Kp7-6 and concanamycin A. Data are presented as the mean±s.e.m. (NS; * P <0.05, *** P <0.001, one-way ANOVA with Tukey post hoc test). ( c ) VM DA neuron survival with SIINFEKL, OT-1 cells pre-pulsed with SIINFEKL and microglial medium previously exposed to LPS, α-syn or NM. Data are presented as the mean±s.e.m. (NS; * P <0.05, ** P <0.01; *** P <0.001, one-way ANOVA with Tukey post hoc test). Each experiment was repeated at least in triplicate and within each experiment, each condition was also performed at least three times. For each condition, neurons on n =24 fields at × 20 were quantified. ConA, concanamycin A; CTRL, control; IFN, interferon gamma; NS, nonsignificant; SIIN, SIINFEKL; Veh, vehicle. Full size image We then explored the mechanism of induced neuronal death by CTLs. We found that the Fas/Fas ligand antagonist, Kp7-6, the caspase inhibitor, Z-VAD-FMK, and the perforin/granzyme antagonist, concanamycin A, each protected against CTL-mediated neuronal death, and that the combination of Kp7-6 and concanamycin A completely blocked neuronal death ( Fig. 6b ). These results indicate that both Fas/Fas ligand and perforin/granzyme pathways play a role in SN neuron CTL-mediated death. Finally, as predicted from MHC-I induction by activated microglia ( Fig. 3d ), the combination of SIINFEKL, CTLs and medium conditioned by microglia exposed to LPS, α-syn or NM caused extensive neuronal death ( Fig. 6c ). Thus, SN neuronal MHC-I can be triggered by secretion of IFN-γ from microglia activated by proinflammatory compounds or two substances, NM and α-syn, present in the extracellular milieu of the SN in PD. We propose an immunologically-based mechanism that may link activated microglia, increased cytosolic oxidative stress and neuronal death of catecholamine neurons. Microglia activated by NM, native α-syn, modified α-syn or mutant α-syn release IFN-γ that in turn induce MHC-I expression in neurons. Catecholamine neurons may be subject to additional oxidative stress due to the presence of cytosolic DA, and this could lead to their MHC-I induction. The capacity of catecholamine neurons to process and display antigens may render them selective targets for T-cell-mediated cell death. Although CNS neurons have been classically considered ‘immunoprivileged’ and to not present antigen, several studies have identified neuronal MHC-I expression in rodents [3] , [5] , [7] , [9] , [10] , [11] , [12] , [14] , [15] . We provide, to our knowledge, the first data demonstrating that human adult SN and LC neurons express MHC-I, as confirmed by a variety of approaches. First, we detected immunolabel for both MHC-I subunits, HLA and β2m, in SN and LC neurons by fluorescent, histochemical and electron microscopic means. Second, we identified mRNA for both subunits in laser-captured SN NM-containing neurons. Third, using mass spectrometry, we identified β2m and specific HLA alleles both in isolated NM organelles and purified NM from organelles and tissues. The human population expresses thousands of HLA-A, B and C alleles [48] , and remarkably, in samples of isolated NM organelles and purified NM obtained from a single subject’s SN, mass spectrometry identified peptides that indicate the expression of specific HLA-A, HLA-B and HLA-C alleles ( Table 1 ). We thus find that a subset of adult human neurons express MHC-I. In agreement with previous studies [21] , [22] , [23] , we did not observe the presence of neuronal MHC-I or β2m in other regions of the adult brain examined including cortex, hippocampus or striatum. Human stem cell-derived DA neurons that exhibit properties of SN DA neurons [28] were also induced to express MHC-I by human IFN-γ, a response analogous to that of mouse neurons. Thus, multiple lines of independent data demonstrate that human neurons, in particular catecholamine neurons, possess the ability to express MHC-I in their cell membrane. When the expression of HLA in TH + neurons was compared in postmortem samples from control versus PD individuals, we observed that the proportion of HLA + in SN and LC neurons was higher in control than in pathological specimens ( Fig. 1e,f ). This would be expected if neurons that were HLA + were selectively destroyed over the course of the disease. We stress, however, that the results must be interpreted cautiously, as the initial proportion of HLA + cannot be ascertained, nor can the duration that human neurons express the protein. In many cases, moreover, the total number of surviving NM + /TH + neurons, especially in the LC PD sections, was very low and unlikely to reflect the proportion during early disease stages. It is further possible that the presence of HLA in human catecholamine neurons is related to another biological process and not to antigen presentation. We identified an association of MHC-I and NM organelles by mass specrometry and immunolabel. NM organelles are autophagic lysosomes that trap and concentrate cytosolic and organelle proteins, and NM synthesis is induced by cytosolic DA [24] . These lysosomal compartments may participate in neuronal antigen presentation, either as an alternative to or following proteasomal processing [1] , [49] . New work demonstrates roles for autophagic lysosomes in the MHC-I response to bacterial infection [50] , suggesting that uptake into lysosomes may participate in the normal handling and degradation of the protein. Consistent with previous studies [3] , [14] , [15] , we found that cultured murine neurons from multiple regions (VM, LC, cortex, striatum, thalamus) could be induced to display MHC-I. Our data demonstrate that catecholamine neurons of the VM and LC were the most responsive to MHC-I induction. L-DOPA, which is converted to cytosolic DA in SN and LC neurons, triggered MHC-I expression, consistent with a role for oxidative stress in enhancing MHC-I [38] via cytosolic catecholamine oxidation. It may be that the presence of cytosolic catecholamine is responsible for the particular presence of MHC-I in human SN and LC catecholamine neurons. We note that these findings should not be construed as suggesting that L-DOPA should not be used clinically; the high exposures used in this study are intended to load the cytosol with high DA levels and not to emulate therapeutic L-DOPA exposure in patients with PD. Additional oxidative stress in LC and SN neurons may result from tonic neuronal firing activity driven by L-type calcium currents [44] , [51] . Our results with OT-I T cells indicate that neuronal death ensues when neuronal MHC-I is expressed and displays a specific antigen recognized by a specific CTL. Previous studies of neuronal killing by CTLs [14] , [15] used exogenous short viral and OVA-derived peptides in culture. We report that VM DA neurons can internalize and present foreign antigen, as addition of the large precursor protein OVA to VM cultures induced SIINFEKL-MHC-I expression on the plasma membrane and within neuronal cytosol. This neuronal MHC-I is immunologically competent, as demonstrated by the induction of CTL proliferation and both Fas and perforin-based CTL neuronal killing. While the loading of peptide onto MHC-I can apparently occur in neurons as well as extracellularly, proteolytic processing of the OVA might occur in non-neuronal compartments, including in astrocytes or by extracellular proteases. There is a general consensus that many neurodegenerative diseases induce a robust inflammatory response, but it remains unclear how this inflammatory response is related to chronic neurodegeneration. Our results suggest a selective upregulation of neuronal MHC-I, antigen presentation and cytolytic activity that may participate under some pathophysiological conditions. It has recently been demonstrated that microglia can be activated by substances released by degenerating neurons in PD, such as α-syn [34] , [52] or NM [35] , [53] , and that activated microglia can elicit neurotoxic responses [54] , [55] , [56] . Both NM and α-syn are found extracellularly in the postmortem brain of PD patients [57] , a disorder that features high levels of activated microglia in the SN [33] and high levels of intracellular oxidative stress [39] . PD patients are reported to possess CNS chemotactic signals [58] and a compromised blood brain barrier [59] , [60] , which may explain why CTLs are found at substantially higher numbers in the CNS of PD patients than in age-matched controls [27] . Catecholamine neuronal display of antigenic MHC-I could participate in a range of additional neurological disorders. For example, Japanese encephalitis virus can induce MHC-I expression in non-neuronal cells by interferon type 1 [61] , whereas in mice, IFN-γ plays a role in paraquat-induced neurodegeneration involving oxidative and proinflammatory pathways [62] . CNS-directed expression of IFN-γ produces basal ganglia calcification and nigrostriatal degeneration [63] . In human case studies, a link is described between chronic hepatitis C patients who were treated with type 1 interferon and developed PD-like symptoms that reversed when the treatment was halted [64] . Thus, both clinical reports and the present results suggest reason to further explore roles for activated microglia, antigen presentation, neuronal MHC-I expression and recruitment of CTLs in neurodegenerative diseases, including PD, that feature the presence of T cells, activated microglia, intracellular oxidative stress and aggregates of α-syn in the SN and LC. Tissue obtaining and handling This study was approved by the Institutional Review Board of the Institute of Biomedical Technologies – National Research Council of Italy (Segrate, Milano, Italy), the New York Brain Bank (Columbia University) and the Center for Neurologic Diseases (Harvard Medical School). Informed consent was obtained from all subjects. Brain samples from 26 normal subjects and 9 PD patients were obtained during autopsy within 5–42 h after death of male and female subjects without evidence of neuropsychiatric and other degenerative disorders. At histological examination, control samples showed no macroscopic neurological, vascular alterations, Lewy bodies or other pathological markers. Tissues from PD subjects were examined histologically by routine staining to confirm loss of SN and LC pigmented neurons, the presence of Lewy bodies and extraneuronal NM. Subjects ages were between 47 and 94 years old, and each PD sample was paired with an age-matched control. Samples from eight control and nine PD individuals were used for immunohistochemistry and immunofluorescence; samples from one control subject was used for electron microscopy; samples from eight control subjects for mass spectrometry; two existing laser-captured microdissected microarray data sets of 17 controls were analyzed for mRNA expression. Each experiment described below was performed at least in triplicate. Immunohistochemistry and immunofluorescence SN/VTA, LC, hippocampal with adjacent entorhinal cortex and striatum (caudate) tissues blocks for histology and histochemistry were fixed in 10% formalin (pH 7.2–7.4) and embedded in paraffin [65] . Tissue sections were incubated with citric acid at 95 °C for 30 min to retrieve antigen and blocked in normal serum; those sections designated for immunohistochemistry were treated with H 2 O 2 to inactivate endogenous peroxidase. Primary antibodies for immunohistochemistry and immunofluorescence were the following: for human MHC-I, we used a mouse monoclonal antibody raised against amino acids 63–362 of the human HLA, 1:100, Santa Cruz Biotechnology (catalogue number: sc-55582; this epitope is shared by HLA-A, HLA-B and HLA-C and so detects all three), and β2m (mouse monoclonal antibody raised against amino acids 1–120 of the human β2m, 1:100, Santa Cruz Biotechnology, catalogue number: sc-13565). A second antibody against human β2m was used (mouse monoclonal antibody raised against amino acids 1–119 of human β2m, 1:100, Abnova, catalogue number: H00000567-M01), that provided the same pattern of staining as the HLA and the original β2m antibodies. For human MHC-II: a mouse monoclonal antibody raised against HLA-DR/DP/DQ/DX (CR3/43), 1:100, Santa Cruz Biotechnology, catalogue number: sc-53302. For TH: rabbit polyclonal, 1:2,000, Millipore, catalogue number: AB152. For Fox-3: rabbit polyclonal, 1:500, Abcam, catalogue number: ab104225. For CD8 + : rabbit polyclonal, raised against a synthetic peptide sequence comprising the 13 C-terminal amino acids of the cytoplasmic domain of α-chain of the CD8 molecule, 1:50, Thermo Scientific, catalogue number: RB-9009-P1. Preliminary control experiments in which the primary antibodies were omitted or HLA (A, B and C) and β2m antibodies were pre-adsorbed with the corresponding neutralizing peptide (293T cell lysate transfected with the sequence corresponding to the HLA epitope shared by HLA (A, B and C) and human full-length β2m peptide, respectively), were performed to confirm the specificity of the primary antibodies ( Supplementary Fig. 4A ). The HLA (A, B and C) and β2m primary antibodies produced a pattern of label similar to well-established MHC-I + structures in human. The immunolabel of blood vessels within the same sections was used as an internal positive control to confirm that the labelling techniques were successful. As the pre-adsorption control does not prove that the monoclonal antibody does not bind another protein, but rather that it binds to the protein of interest, additional controls for HLA and β2m primary antibodies were carried out. From one control brain, the SN of the opposite hemisphere that was processed for immunostaining was homogenated for western blots. Both antibodies produced a single, clear band that matched with the appropriate molecular weight (46 KDa for HLA and 12 KDa for β2m, see Supplementary Fig. 4B,C ). As an additional control for CD8 + antibody, human spleen (paraffin sections obtained from Cell Marque) was used to test specificity of this antibody, as well as absence of labelling when omitting the primary antibody ( Supplementary Fig. 4D ). Sections designated for immunohistochemistry were incubated with a biotinylated secondary antibody (1:200, VectorLabs) followed by avidin–biotin complex (VectorLabs); V-VIP was used as the chromogen (VectorLabs). Sections designated for immunofluorescence were incubated with secondary fluorescent antibodies (Alexa Fluor-488 or Alexa Fluor-594, 1:400, Invitrogen) and mounted with a water-based medium. Images were captured with a Leica SP5 microscope. There was no fluorescence bleedthrough of secondary antibodies under the conditions used. Counting of NM + , TH + and HLA + neurons was performed in three sections per patient ( n =8 or 9 patients per condition) using a fluorescent microscope at × 20 magnification. Quantification was on the basis of the absolute presence of HLA and rated as positive or negative. Electron microscopy Immunoelectron microscopy experiments were carried out on tissue blocks fixed in 4% paraformaldehyde/0.25% glutaraldehyde in cacodylate buffer (0.12 M, pH 7.4) and embedded in LRW resin. Ultrathin sections were incubated with an HLA (A, B and C) antibody (1:200, Santa Cruz Biotechnology) and then with a gold particle (15 nm)-conjugated secondary antibody (1:100, British Biocell International). Micrographs were acquired by a transmission electron microscope LEO 912 (Advanced Light and Electron Microscopy BioImaging Center – San Raffaele Scientific Institute). Mass spectrometry MHC-I peptides were identified by mass spectrometry in NM pigment isolated from SN, organelles containing NM, and NM separated from organelles obtained as reported [25] . Digested peptides were separated by two-dimensional micro-liquid chromatography coupled to an ion trap mass spectrometer (2DC-MS/MS). The SEQUEST database search algorithm was used to match experimental spectra to peptide sequences in the database. Peptide search was executed against an updated non-redundant human protein sequence database and MHC-I isoform (HLA gene) database from National Center for Biotechnology Information (NCBI) ( www.ncbi.nlm.nih.gov ). Laser capture microdissection and bioinformatics analysis Affymetrix CEL files for the National Brain Databank data set (NBD) were normalized to ‘all probe sets’ using standard procedures, and scaled to 100 by the MAS5 algorithm implemented in the Bioconductor package [26] , [66] . Laser-capture microdissection and microarray methods used to generate the NBD data sets described [67] . Western blotting Tissue for western blotting was obtained from the New York Brain Bank frozen, and then rapidly homogenated at 4 °C in lysis buffer containing 50 mM of Tris-HCl, 150 mM of NaCl, 5 mM of EDTA and 1% of Triton-Tx. Protein concentration of the total homogenate was measured using the BCA assay (Thermo Scientific). A total of 60 μg of protein per lane were run on a 10% polyacrylamide gel for HLA antibody and on a 15% polyacrylamide gel for β2m antibody. Proteins were transferred to PVDF membranes (Immobilon, Millipore, Bedford, MA, USA). After blocking in 5% dry milk, primary antibodies were applied overnight at 4 °C, then rinsed three times in Tris-buffered saline containing 0.1% Tween-20 (Fisher Scientific). Peroxidase-labelled secondary antibodies were applied for 1 h at RT, blots rinsed in Tris-buffered saline-Tween as before, developed with enhanced chemiluminescence (Immobilon HRP substrate reagents, Millipore), and then exposed to film (Crystalgen). HLA (1:100, from Santa Cruz Biotechnology) and β2m (1:100, from Abnova) primary antibodies were used. Actin (1:500,000, from Sigma-Aldrich) primary antibody was used as a loading control. hES-derived DA neuronal cultures hES-derived DA neuronal cultures were obtained as described [28] . Briefly, H9 human ES cells were subjected to dual SMAD-inhibition followed by exposure to sonic hedgehog, purmorphamine, FGF8 and CHIR99021. Neurons were passaged on day 20, replated on glass-bottom dishes on day 30 at a density of 200,000 cells per 20 μl droplet, and then matured in Neurobasal media with the addition of B27 supplement, GDNF, BDNF, ascorbic acid, cAMP, TGFbeta and DAPT. hES-derived spinal MN cultures expressing EYFP under control of the human synapsin promoter were generated by exposure to dual SMAD-inhibition followed by caudalization with retinoic acid and ventralization through the hedgehog pathway. MN aggregates were replated on day 20 and matured in Neurobasal media with the addition of B27 supplement, GDNF, BDNF, ascorbic acid, cAMP and DAPT. Cultures were treated with human IFN-γ (eBioscience) at a nontoxic concentration for hES (100 ng ml −1 , 72 h). Cultures were then incubated with the MHC-I antibody before fixation in 4% paraformaldehyde and double immunofluorescence for TH and MHC-I as above. Micrographs were acquired using a Leica TCS SP5-II inverted confocal microscope. Mice Animal protocols were approved by the Columbia University Institutional Animal Care and Use Committee and in accordance with the National Institutes of Health Guide to the Care and Use of Laboratory Animals guidelines. Mouse lines including wild-type C57BL/6, OT-1, OT-2 and B6.129P2-B2mtm1Unc/J mice were maintained under pathogen-free conditions and had access to food and water ad libitum. Each experiment described below was performed at least in triplicate. Primary cultures Primary cultures of microglial cells, SN, VTA, VM (including SN and VTA), LC, cortical, striatal and thalamic neurons were derived from brains of newborn C57/Bl6 or B6.129P2-B2m tm1Unc /J mice (0–3 days, either sex) [31] . B6.129P2-B2m tm1Unc /J mice were generated by a targeted disruption of the β2m gene, and have little or no MHC-I protein expression on the cell surface [68] . Briefly, for microglial cultures cells dissociated from five cortexes of 0–3 days old C57/Bl6 mice were seeded onto 75 cm 2 cell culture flasks in microglial culture medium (MEM supplemented with calf serum, glucose 45%, penicillin/streptomycin, insulin (25 mg ml −1 ) and 200 mM glutamine) in a 5% CO 2 incubator at 37 °C (ref. 31 ). Two weeks later, microglia were detached from flasks by mild shaking and plated on 12-well plates at a density of 45,000–50,000 microglial cells per well. For neuronal cultures, the area of interest was dissected and neurons were dissociated and plated at a density of 80,000 cm −2 onto a layer of rat cortical glial cells grown on round glass coverslips and maintained in culture medium without added GDNF (glial cell line-derived neurotrophic factor) in a 5% CO 2 incubator at 37 °C for 5–9 days [31] . Primary DCs were obtained from mouse (either sex) femur hematopoietic stem cells. In brief, mouse femur hematopoietic stem cells from bone marrow were harvested from the hind legs of 8–12-week old male wild-type C57BL/6J and plated at 2 × 10 6 cells ml −1 density in DC culture medium (DMEM supplemented with 10% FBS, 1 × non-essential amino acids, 2 mM L-glutamine, 1 mM sodium pyruvate and 20 mM HEPES). For differentiation to dendritic cells, 10 ng ml −1 of recombinant mouse GM-CSF was added to media. Cells were fed every 2 days with fresh DMEM containing GM-CSF, and the cultures were trypsinized after 8 days and plated at 4 × 10 5 cells cm −2 density to be used for experiments the following day [69] . OT-1 CD8 + and OT-2 CD4 + T cell lines, a gift kindly received from Dr Raphael Clynes (Department of Medicine and Microbiology, Columbia University Medical Center), express a transgene encoding T-cell receptor that specifically recognizes SIINFEKL peptide (derived from OVA) bound to MHC-I H-2Kb or to MHC-II I-A/I-E [70] . Activated primary OT-1 and OT-2 T cells were generated by the addition of SIINFEKL to the cultures [58] . Briefly, OT-1/OT-2 mouse spleens were dissected and homogenized, the released cells were pelleted and resuspended in 5 ml ACK buffer (0.15 M NH 4 Cl, 1 mM KHCO 3 , and 0.1 mM EDTA) for 1 min to lyse red blood cells, and the splenocytes were pelleted, washed, resuspended at 5 × 10 6 cells ml −1 in OT-1 growth medium containing 0.75 μg ml −1 SIINFEKL peptide, and incubated at 37 °C in a 95% air/5% CO 2 humidified atmosphere. On days 3 and 5, 25 ml of fresh OT-1/OT-2 growth medium containing 10 U ml −1 of mouse recombinant IL-2 was added to the cultures. On day 7, the cells were harvested and OT-1/OT-2 cells were purified by centrifugation at 400 g for 30 min at room temperature over a Histopaque gradient (density=1.083) [47] . Cellular treatments IFN-γ (R&D Systems) was used at a range of nontoxic concentrations for neurons or OT-1 cells (10 pg ml −1 –100 ng ml −1 , 72 h). 12-well cell culture plates were pre-treated with LPS (500 ng ml −1 , Sigma-Aldrich), NM (5 μg ml −1 ), α-syn, Nit-α-syn or Mut-α-syn (200 μg ml −1 , kindly provided by Peter Lansbury, Harvard University) for 72 h before plating 45,000–50,000 microglial cells per well for an additional 24 h. A neutralizing IFN-γ antibody (1:500, PBL InterferonSource) was used to block IFN-γ released from microglia. VM neurons were incubated for 72 h with microglial medium pre-stimulated by LPS, NM, α-syn, Nit-α-syn or Mut-α-syn. As a control experiment, we directly incubated VM neurons with the same compounds in the absence of microglia. In another set of experiments, VM, cortical and striatal primary neurons were incubated for 72 h with microglial medium pre-stimulated by LPS, NM, α-syn. NM was induced in SN-cultured neurons by using L-DOPA [24] (Sigma-Aldrich). For foreign protein processing and subsequent antigen presentation, VM cultures were maintained for 7 days in either (1) BSA/serum-free neuronal medium, (2) BSA/serum-free supplemented with OVA (2.5 mg ml −1 ), adding IFN-γ (100 ng ml −1 ) or saline for an additional 72 h. ELISA The concentration of IFN-γ released by microglia (plated as above) was measured by an ELISA kit (eBioscience) that detected the amount of this proinflammatory cytokine in a range of 0.7–100 pg ml −1 . Immunofluorescence Cell cultures were double-labeled for MHC-I using a specific antibody raised against the H-2K b and H-2D b class I alloantigens (mouse monoclonal, 1:100, BD Biosciences, catalogue number: 553575), MHC-II (by using a mouse monoclonal antibody that reacts with a polymorphic determinant shared by the I-A[b], I-A[d], I-A[q], I-E[d] and I-E[k] MHC-II alloantigens, 1:100, BD Biosciences, catalogue number: 556999) or SIINFEKL-MHC-I (mouse monoclonal, 1:100, eBioscience, catalogue number 14-5743-81) and TH (rabbit polyclonal, 1:2,000, Millipore, catalogue number: AB152) or MAP-2 (rabbit polyclonal, 1:1,000, Millipore, catalogue number: AB5622), fixed with freshly prepared 4% paraformaldehyde (Electron Microscopy Sciences), blocked with normal serum (Jackson Immunoresearch) and incubated with fluorescent secondary antibodies (Alexa Fluor-594 or Alexa Fluor-488, 1:400, Invitrogen). Images were captured using a Leica SP5 microscope system. There was no fluorescence bleedthrough of secondary antibodies under the conditions used. MHC-I label observed in the neuronal cultures obtained from wild-type mice was absent in neurons from β2m KO mice ( Fig. 3a ). To assess the proportion of TH + and MAP-2 + neurons that expressed MHC-I + , first TH + and MAP-2 + neurons were counted in 24 fields surrounding the border of the well at × 20 magnification. The number of TH + or MAP-2 + neurons with intact soma and two or more neurites equal to or greater than the diameter of the cell soma was counted. Then, the fluorescent filter was inserted for each field to determine how many of these neurons also expressed MHC-I. To further analyze the specificity of the MHC-I antibody, a western blot was run of wild-type versus β2m KO brain tissue (see western blot paragraph below for detailed method). A single band (~30 KDa) was observed in lanes loaded with brain tissue from wild-type mice, whereas there were no visible bands in the lanes that contained brain tissue from β2m KO. A positive control (mouse spleen homogenate) displayed a band at the same molecular weight ( Supplementary Fig. 4E ). Western blotting The brains of three C57/BL6 and three B6.129P2-B2m tm1Unc /J were dissected on ice and then rapidly homogenated at 4 °C in lysis buffer containing 50 mM of Tris-HCl, 150 mM of NaCl, 5 mM of EDTA and 1% of Triton-Tx. Protein concentration of the total homogenate was measured using the BCA assay (Thermo Scientific). A total of 20 μg of protein per lane were run on a 12% polyacrylamide gel. Proteins were transferred to PVDF membranes (Immobilon, Millipore Corporation, Bedford, MA). After blocking in 5% dry milk, primary antibody (MHC-I antibody raised against the H-2K b and H-2D b class I alloantigens, mouse monoclonal, 1:100, BD Biosciences), was applied overnight at 4 °C, then rinsed three times in Tris-buffered saline containing 0.1% Tween-20 (Fisher Scientific). Peroxidase-labelled secondary antibodies were applied for 1 h at RT, blots rinsed in Tris-buffered saline-tween as before, developed with enhanced chemiluminescence (Immobilon HRP substrate reagents, Millipore), and then exposed to film (Crystalgen). Actin (1:500,000, from Sigma-Aldrich) primary antibody was used as a loading control. A total of 20 μg of mouse spleen homogenate was loaded as a positive control for the MHC-I antibody. Proliferation and killing assays OT-1 CD8 + cell proliferation was assessed by BrdU incorporation. For OT-1 T-cell cytotoxicity assays, DC and VM (from C57BL/6 and B6.129P2-B2mtm1Unc/J mice) cell cultures were incubated with neuronal medium or neuronal medium containing 100 ng ml −1 of IFN-γ (R&D Systems). Neurons were loaded with or without SIINFEKL peptide (1 μM), and, subsequently in vitro activated OT-1 cells were added at a density of 100,000 cells per well and co-incubated for 24 h. We used the same conditions for VM cell cultures with microglial medium previously stimulated with LPS, NM or α-syn instead of IFN-γ. Neurons were pre-incubated with IFN-γ and SIINFEKL peptide as above, and then with (1) a pan-caspase general inhibitor (Z-VAD-FMK, 20 μM, 24 h, IMGENEX); (2) a specific granzyme/perforin inhibitor (concanamycin A, 100 nM, 24 h, Sigma-Aldrich); (3) a specific Fas/FasL antagonist (Kp7-6, 1 mM, 24 h, EMD Biosciences) and (4) concanamycin A and Kp7-6 together. OT-1 cells were then added to the culture (100,000 cells per well) and maintained for 24 h. Following immunocytochemical staining of VM neurons, we assessed the proportion of surviving DA (TH + ) and non-DA cells (MAP-2 + , TH − ). Total numbers of TH + and MAP-2 + neurons were counted in 24 fields surrounding the border of the well at × 20 magnification. The number of surviving TH + neurons with an intact soma and two or more neurites equal to or greater than the diameter of the cell soma was counted and normalized to the number in untreated cultures. Statistics Results are presented as mean±s.e.m. Each experiment was repeated at least three times, and each condition was also examined in three subjects or cultures within each experiment. Two-way ANOVA was used to analyze the IFN-γ dose-response experiments. Two-tailed Student’s t -test (or Man–Whitney U -test for nonparametric cases) or one-way ANOVA with Tukey post hoc tests were used to analyze the other experiments. How to cite this article: Cebrián, C. et al . MHC-I expression renders catecholaminergic neurons susceptible to T-cell-mediated degeneration. Nat. Commun. 5:3633 doi: 10.1038/ncomms4633 (2014). Accession Code: The National Brain Databank (NBD) microarray data set is publicly available in the National Brain Databank database under the accession name ‘Parkinson’s’.